Revealing letters in rolled Herculaneum papyri by X-ray phase-contrast imaging Hundreds of papyrus rolls, buried by the eruption of Mount Vesuvius in 79 AD and belonging to the only library passed on from Antiquity, were discovered 260 years ago at Herculaneum. These carbonized papyri are extremely fragile and are inevitably damaged or destroyed in the process of trying to open them to read their contents. In recent years, new imaging techniques have been developed to read the texts without unwrapping the rolls. Until now, specialists have been unable to view the carbon-based ink of these papyri, even when they could penetrate the different layers of their spiral structure. Here for the first time, we show that X-ray phase-contrast tomography can reveal various letters hidden inside the precious papyri without unrolling them. This attempt opens up new opportunities to read many Herculaneum papyri, which are still rolled up, thus enhancing our knowledge of ancient Greek literature and philosophy. The explosion of Vesuvius in 79 AD, the most famous eruption of this volcano [1] , destroyed several Roman towns in Campania, especially Pompeii and Herculaneum. The eruption buried these sites under very thick layers of volcanic material, preserving them in what became an exceptional opportunity for students of ancient Greco-Roman culture. After initial, sporadic discoveries by well-diggers and treasure hunters, Charles, the Bourbon King of Naples, ordered that they be explored in what became the first systematic archaeological excavations [2] , [3] , [4] , [5] . After a first discovery of papyrus rolls in 1752 (ref. 6 ), in 1754 (refs 5 , 7 , 8 ), from late February through August, an entire library was discovered in a small room of a huge villa (thought by some to have belonged to the wealthy Roman statesman Calpurnius Piso Caesoninus [9] ) containing hundreds of handwritten carbonized papyrus scrolls carefully stored in shelves covering its walls. This rich book collection, consisting principally of Epicurean philosophical texts, is a unique cultural treasure, as it is the only ancient library to survive together with its books. The texts preserved in these papyri, now mainly stored in the Officina dei Papiri in the National Library of Naples [10] , had been unknown to scholars before the discovery of the Herculaneum library, since they had not been copied and recopied in late Antiquity, the middle ages and Renaissance. A quite sophisticated mechanical method for unrolling the best preserved scrolls—applicable to their final, interior parts that are less than a third of their original length—dreamed up in 1754 by Antonio Piaggio [2] , [3] , [4] , [5] continued to be used until the beginning of the 20 th century on those scrolls that could in principle withstand the physical stress imposed by the process. Different opening techniques, all less effective, have been tried over the years [11] until the so-called ‘Oslo method’ was applied in the 1980s on two Herculaneum scrolls now in Paris [12] with problematic results, since the method required the rolls to be picked apart into small pieces [13] . All further attempts to unroll the papyri or to separate their layers mechanically had been abandoned until now to preserve their physical integrity and the possibility of reading them as continuous texts one day, because an excessive percentage of these ancient texts was irretrievably lost by the application of such methods. On the other hand, in the last 20 years a great deal of progress has been made in reading the Herculaneum texts that had already been unrolled. In particular, the use of binocular microscopes, and digital photography, employing ‘multispectral’ filters that isolate a narrow portion of the near-infrared spectrum, have both improved the readability of these texts considerably [14] , [15] . Unfortunately, these techniques are not applicable to texts that remain rolled-up due to the superposition of papyrus layers and the weak penetration of most types of radiation exploited by multispectral techniques. In Antiquity, papyri were written using a black carbon-based ink obtained from smoke residues, the density of which is almost the same as that of the carbonized papyrus. Until now, therefore, it has appeared impossible to distinguish ink from papyrus inside a papyrus roll using the penetrating radiation of a conventional X-ray source and technique, where the X-ray image contrast is based exclusively on the X-ray-absorption patterns of different materials [16] . The X-ray fluorescence imaging method has been successfully applied to the chemical mapping of writings in ancient manuscripts and palimpsests that are covered by other writings, paintings or mold, for example [17] . However, to read the writing on surfaces hidden within papyrus scrolls or on layers of fragmentary rolls below their exposed upper surfaces, a different technique is needed—one that discriminates modifications inside the scrolls. In X-ray computed tomography (XCT), which has become a conventional tool with broad applications in medicine, materials science, palaeontology and archaeology, as well as several industrial areas, the image contrast mechanism is based on differential X-ray absorption within a compound object. This technique works particularly well for discriminating strongly absorbing materials, such as bone, from weakly absorbing materials such as soft tissues [18] . However, many important applications in biology, medicine and even materials science require the detection of absorption variations between weakly absorbing (low-Z) materials, like the ink of the Herculaneum scrolls and its papyrus support. As the variations in this case are minimal, XCT does not appear to be a suitable technique, but one promising approach that has proven to overcome these limitations is the X-ray phase-contrast tomography (XPCT) technique [19] . Unlike XCT, XPCT exploits variations in the refractive index (that is, X-ray phase shifts) between structures that absorb quite uniformly within a composite object, thus significantly enhancing the image-contrast effect. More precisely, in propagation-based phase-contrast imaging (PBI), quasi-coherent radiation illuminates the object producing a spatially variant phase shift of the X-ray beam [20] , [21] . As the X-rays propagate from the sample, portions of the wavefront that have experienced different deflections in the sample generate characteristic patterns. Due to Fresnel diffraction, the phase shifts are transformed into measurable intensity variations, which are recorded by a detector located at an appropriately chosen distance. Over the last 15 years, phase-contrast imaging has undergone rapid progress, and various methods aimed at obtaining the phase information have been developed. In the literature, several articles [22] , [23] , [24] , [25] , [26] , [27] show the suitability of this technique for discriminating different materials of similar composition within a single object, as in the case of black charcoal ink and carbonized papyrus. Here we examine two of the six Herculaneum scrolls (one unrolled and the other still rolled-up) presented as a ‘gift’ to the Premier Consul Napoléon Bonaparte in 1802 and currently belonging to the collection of the Institut de France . The first sample is a fragment of the unrolled scroll, PHerc.Paris. 1 , while the second ( PHerc.Paris. 4 ) is an (almost) entire rolled-up scroll. Our results show that XPCT is the first non-destructive technique that enables us to read many Greek letters and some words in the interiors of rolled-up Herculaneum papyri without impairing their physical integrity, as the previous unrolling techniques had done. This is extremely important because the fragility of carbonized papyri requires the most careful manipulation. Sample characteristics The Herculaneum scrolls were burnt by a blast of furnace-like (c. 320 °C) gas from the volcano into a vastly homogenous sample matrix. In Antiquity, the most common writing material used for books and other documents was papyrus. The stalks of papyrus plants were cut into thin strips, then two strips were laid atop and perpendicular to one another; these strips were then combined by pressing them until the plant’s natural starch that acted as a paste. The resulting sheets of papyrus were then smoothed and bleached. A papyrus roll consisted of some number of such sheets pasted together end on end. The resulting sheet, which could reach 15 m or more in length, was then rolled up from right to left, so that it could be read from left to right. Papyrus writing material, therefore, consisted of two layers, whose fibres ran perpendicular to one another; the scribe would usually write the text in vertical columns on the side of the papyrus sheet where the horizontal fibres were uppermost. The carbon-based ink he used did not penetrate into the papyrus fibres, but sat atop them. As we shall see, this fact proved to be crucial for our experiments. In general, the letters stand out in slight relief from the papyrus surface, a phenomenon that is familiar to papyrologists reading unrolled Herculaneum texts with the aid of a microscope. It is precisely this morphological feature that allows the highlighting of letters by XPCT, although the difference between ink composition and carbonized papyrus is not sufficient to enhance any differential absorption using conventional XCT. The relief of the letters, which rise at least one hundred microns above the surface of the papyrus fibres, is by itself sufficient to produce appreciable phase contrast. Writing detection in a fragment of papyrus scroll PHerc.Paris. 1 To prove the effectiveness of the proposed technique, a first experiment was performed on a very small part of fragment 101 from PHerc.Paris. 1 , removed from the roll thanks to an ‘unrolling’ operation conducted by the Oslo method in Naples in 1986/7, and showing several superposed layers of papyrus. On one of the hidden layers, we have succeeded in reading two words in successive lines. In Fig. 1a the sequence of Greek capital letters ΠIΠTOIE( pi-iota-pi-tau-omicron-iota-epsilon ), could be read either as ππτOιε[ν or as ππτOι followed by a word beginning with an epsilon , for example, [ν (or ε[ισ), and meaning ‘would fall’. In the following line ( Fig. 1b ), it is possible to read another letter sequence, almost certainly EIΠOI ( epsilon-iota-pi -omicron-iota ), meaning ‘would say’. The spatial resolution of the detector (see Methods) is 100 microns so that the letters observed in this papyrus, which are about 2–3 mm, are fully disclosed by the imaging process. 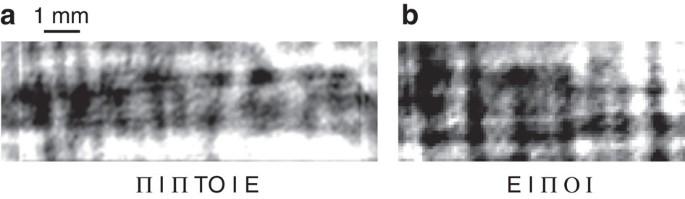Figure 1: Two words read on a hidden layer of the fragmentPHerc.Paris. 1fr. 101. (a) The sequence of Greek capital letters ΠIΠTOIE (pi-iota-pi-tau-omicron-iota-epsilon); (b) The letter sequence of the next line, EIΠOI (epsilon-iota-pi-omicron-iota). Figure 1: Two words read on a hidden layer of the fragment PHerc.Paris. 1 fr. 101. ( a ) The sequence of Greek capital letters ΠIΠTOIE ( pi-iota-pi-tau-omicron-iota-epsilon ); ( b ) The letter sequence of the next line, EIΠOI ( epsilon-iota-pi-omicron-iota ). Full size image Writing detection in papyrus scroll PHerc.Paris. 4 The main object of our investigation has been a nearly complete scroll that is typical of rolled-up Herculaneum papyri. This specimen is relatively well preserved and is inventoried as PHerc.Paris. 4 ( Fig. 2a ). In Fig. 2b three orthogonal slices of the reconstructed volume ( Fig. 2c ) give a picture of the morphology of this scroll. The tremendous pressure of the pyroclastic material compressed the scroll and deformed its internal spiral structure, the layers of which are folded in a nearly chaotic and badly entangled fashion. Moreover, in many places the whorls have adhered to one another. Therefore, it should be emphasized that the letters (which were capital letters in all the literary papyri) may be more or less distorted, since they lie on highly non-planar surfaces that are cut by selected planar sections for rendering purposes. All this makes data analysis a challenge, since it is necessary to ascertain the phase contrast associated with the text on a surface, the shape and topology of which exhibit an extremely high degree of complexity. Nevertheless, we were able to discern evidence of this contrast in the reconstruction. 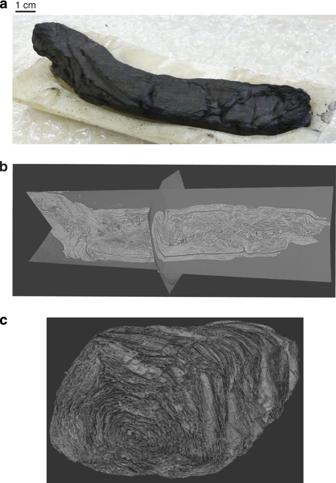Figure 2: The Herculaneum papyrus scrollPHerc.Paris. 4. (a) A picture of thePHerc.Paris. 4lying in its transport holder, fabricated by means of a three-dimensional scan of the external papyrus shape profile (~16 cm length). The carbonized papyrus is extremely fragile. Its deformation was caused mechanically by the eruptive material; (b) three orthogonal slices, and (c) a volume rendition of the reconstructed papyrus, which highlights the huge complexity inside the scroll, where the papyrus convolutions were exposed to tremendous stresses. Figure 2: The Herculaneum papyrus scroll PHerc.Paris. 4 . ( a ) A picture of the PHerc.Paris. 4 lying in its transport holder, fabricated by means of a three-dimensional scan of the external papyrus shape profile (~16 cm length). The carbonized papyrus is extremely fragile. Its deformation was caused mechanically by the eruptive material; ( b ) three orthogonal slices, and ( c ) a volume rendition of the reconstructed papyrus, which highlights the huge complexity inside the scroll, where the papyrus convolutions were exposed to tremendous stresses. Full size image In Fig. 3a , it is possible to make out three letters in linear sequence. The first is undoubtedly an A ( alpha) and the third an N ( nu ). The middle letter, however, requires a more careful interpretation: the loop, which we believe is its topmost part, evokes a P ( rho ), that is, a letter equivalent to English R. We would then have the sequence ‘APN’, which can either come from a single word like αρν-εĩσθαι ‘to deny’ or be divided into the two-letter sequence ‘AΡ’ and the single letter ‘N’, giving, for example, the particle [γ]αρ, ‘for’ (which is always in second position in a clause or sentence) and preceding a word starting with N. In Fig. 3b , the sequence of letters HEY ( êta-epsilon-upsilon ), equivalent in English to a long E followed by the syllable EU, is clearly identified. This sequence falls naturally into the single letter H and the two-letter sequence EU, the former being presumably the feminine definite article ‘the’ and the latter the first syllable of a nominal ( cf. for example, in English euphonia , euphonic ). In Fig. 3c , we can identify the sequence KI, κι ( kappa-iota ), found, for example, in the words of the verb family κινεν ‘to move’. Unfortunately, the risk of confusion is always possible when dealing with horizontal or vertical traces, since they can correspond either to actual letters or to fibres in the papyrus material. The only clearly distinct marks in such a document are rounded or oblique traces, shapes that are not easily confused with papyrus fibres, which run vertically and horizontally, and are therefore letters or parts of letters. Hence, the following letters are relatively easy to distinguish: A, B, Δ, E, Z, Θ, K, Λ, M, N, O, P, C, Υ, Φ, X, Ψ and Ω; while Γ, H, I, Ξ, Π and T are more easily confused. The script here is noticeably different from that of PHerc.Paris. 1 , shown in Fig. 1 . 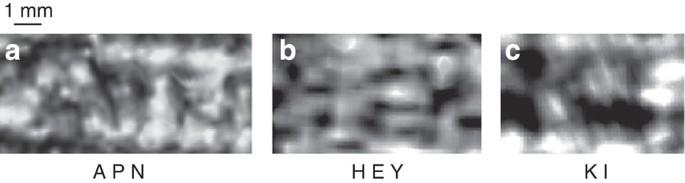Figure 3: The letters discovered insidePHerc.Paris. 4. (a) The sequence of Greek capital letters APN (alpha-rho-nu); (b) the letters sequence HEY (eta-epsilon-upsilon) and (c) the sequence KI (kappa-iota). Figure 3: The letters discovered inside PHerc.Paris. 4 . ( a ) The sequence of Greek capital letters APN ( alpha-rho-nu ); ( b ) the letters sequence HEY ( eta-epsilon-upsilon ) and ( c ) the sequence KI ( kappa-iota ). Full size image The alphabet of this papyrus that we present in Fig. 4 comes from different images of the scroll acquired during the experimental scans. It is to be read as follows: the 24 letters of the Greek alphabets are arranged in three superimposed lines. Lines 1 and 2 consist of letters taken from several internal regions of the sample (for several letters, line 2 shows a second, slightly different, example we were able to obtain). One should not forget that the letters may be heavily distorted, due to the highly non-planar surfaces on which they lie. Line 3 reproduces the corresponding letters extracted from infrared images of a Herculaneum papyrus ( PHerc. 1471 ) opened previously and preserved in the National Library in Naples, Italy; it contains a work by the Epicurean philosopher Philodemus, ‘On Frank Criticism’, which has been studied in depth by one of the authors of the present article. The letters from PHerc. 1471 are meant to help the reader in recognizing the layout of the letters appearing in PHerc.Paris. 4. 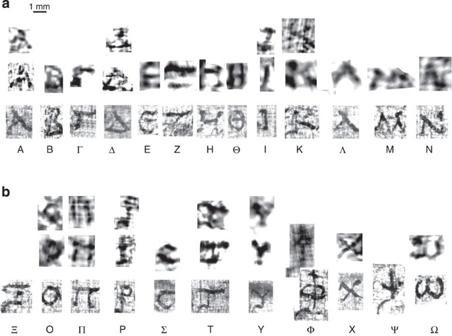Figure 4: The papyrus alphabet fromPHerc.Paris. 4. (a) The alphabet letters from A to N (alphatonu) as revealed by the XPCT experiment, primarily from the innermost region of the papyrus, where the individual coils are more distinguishable, are reported on lines 1 and 2; on line 3 the infrared images of the same letters from the unrolled papyrusPHerc. 1471, which was used as a reference for the writing style of the scrollPHerc.Paris. 4. Printed capital letters of the ancient Greek alphabet are given below line 3. (b) The alphabet letters revealed by the XPCT experiment from Ξ to Ω (xitoomega). Figure 4: The papyrus alphabet from PHerc.Paris. 4 . ( a ) The alphabet letters from A to N ( alpha to nu ) as revealed by the XPCT experiment, primarily from the innermost region of the papyrus, where the individual coils are more distinguishable, are reported on lines 1 and 2; on line 3 the infrared images of the same letters from the unrolled papyrus PHerc. 1471 , which was used as a reference for the writing style of the scroll PHerc.Paris. 4 . Printed capital letters of the ancient Greek alphabet are given below line 3. ( b ) The alphabet letters revealed by the XPCT experiment from Ξ to Ω ( xi to omega ). Full size image In Fig. 4 , PHerc. 1471 was chosen as a reference for comparison with our new alphabet, because some of the letters from the reconstructed specimen PHerc.Paris. 4 show on the left side of their base a small decorative hook that is always present in PHerc. 1471 but is not widespread in the writing style of other papyri in the collection. This does not mean that PHerc.Paris. 4 and PHerc. 1471 were copied by the same hand: we are simply looking at two hands with significant similarities. The alphabet we have reconstructed from PHerc.Paris. 4 lacks only the letters Ξ (English X) and Ψ (English PS); this is not surprising, as these letters are far less frequent as other letters in ancient Greek texts. The overall close similarity of the two hands could lead us to date PHerc.Paris. 4 to the same period as PHerc. 1471 , that is, the second quarter of the first century BC, according to the dating proposed by G. Cavallo [28] . (He characterizes his ‘group M’ as follows: ‘the ductus appears smooth, the lines are subtle, with elegant apexes that give the writing a very refined look. In the treatment of letters, the differences from other Greek writings from Herculaneum (especially group I) are not substantial, but the airy lightness of touch and the light tracing of the apexes, even when they are well marked, generally supply a different stylistic effect. The middle bar of alpha (English ‘A’) is either horizontal or oblique, connected through a loop to the oblique line that descends from right to left (...). Epsilon and theta (the letters ‘E’ and ‘TH’, respectively) usually have a rather short median bar (...). The right stem of êta (a letter form similar to that of English ‘H’) is elegantly arched; the internal oblique strokes of mu (the letter ‘M’) meet in an ample angle, while in some scrolls the outside strokes of mu may be curved or straight and stiff. The letter rho (English ‘R’) extends quite a long way above and below the lines of the writing, while the upsilon (English ‘U’) is almost always bilinear’.) Comparing the alphabet in Fig. 4 with Cavallo’s description of the hands of his ‘group M’, we note an apparent consistency with the writing of PHerc.Paris. 4 . If it is correct to place this hand in Cavallo’s group M, then the papyrus is quite likely to contain a text by Philodemus. Thus, this study, without compromising the physical integrity of the roll, has not merely discovered traces of ink inside it, but has also helped identify with a certain likelihood the style of handwriting used in the text, along with its author. The XPCT used for our experiment has some limitations, since it is not the technique most sensitive to phase variation. It was, however, the best technique to use for this proof-of-concept experiment. In future experiments, further tuning of the PBI technique could improve image quality using a synchrotron beamline with better coherence properties than that used in this proof-of-concept study. On the other hand, another phase-contrast technique, such as grating interferometry [29] , which is sensitive to the derivative of the phase, promises to deliver better contrast and readability of the text’s characters than what might be obtained using PBI, which is sensitive to the Laplacian of the phase. It is extremely difficult to resolve several layers of the innermost windings of the scroll. Since the algorithms available for segmentation fail when applied to a complex surface such as that in Fig. 2 , small continuous portions of the same surface were identified manually in almost all cases. We found lines of more or less clear letters displaying a variable size that is roughly in agreement with the average letter size in the Herculaneum papyri (around 3 mm high). Because of the interwoven geometry of the imperfectly folded scroll, the size of the letters reconstructed by XPCT may vary slightly. The thickness of each of the coils of the spiral making up the papyrus roll is so small as to make selective focus on different areas of the resulting image an extremely delicate matter. This has a significant impact on the reading of confused or blurred letters. Moreover, owing to the complex folding, identifying the parts of the image with particular letters is not always straightforward. Only the asymmetrical letters (such as B, C, K or P) make it possible to know with certainty whether the image shows the letters in the correct, left-to-right, direction of writing. Sometimes the letters appear to be flipped up-down or left-right. Moreover, due to the highly textured nature of the papyrus sheet, a strong phase-contrast signal is present and hides some parts of the characters, which could explain the small number of characters we found. Further integration of the image-segmentation process with tomography will reduce artefacts, such as irregularities and convolution of the reconstructed layers of papyrus. While our first experiments have revealed only small segments of writing and are in need of further refinement, we note that once the XPCT technique has been tuned, the imaging of an entire papyrus scroll should not require more than a few hours of synchrotron beam time that can be obtained by way of a peer-reviewed process. The impact of our discovery that XPCT can read writing inside carbonized papyrus rolls reaches far beyond the study of one particular Herculaneum papyrus. It holds out the promise that many philosophical works from the library of the ‘Villa dei Papiri’, the contents of which have so far remained unknown, may in future be deciphered without damaging the papyrus in any way. This pioneering research opens up new prospects not only for the many papyri still unopened, but also for others that have not yet been discovered, perhaps including a second library of Latin papyri at a lower, as yet unexcavated level of the Villa [30] . Phase-contrast imaging We conducted the experiment at the biomedical beamline ID17 of the European Synchrotron (ESRF, Grenoble, France) in December 2013. The phase-contrast technique used is that of PBI; a scheme of the experimental set-up is in Fig. 5 . The imaging detector was a Fast Readout Low Noise (FReLoN) 2k charge-coupled device camera, and the related optical equipment features a 90 × 90-mm 2 field of view with an effective pixel size of 46 × 46 μm 2 . The scintillator screen used to convert X-rays into visible light consists of a gadolinium oxysulphide layer of 60 μm thickness. The spatial resolution, as measured in such a configuration [31] , is 100 μm in each of the three spatial dimensions and does not depend on the location of the scroll, due to the high number of projections used for tomographic scans. In this first experiment, the sample-to-detector distance was set to ~11 m. The optimum energy of the X-ray beam used was 70 keV (monochromatized by a double-silicon (111) crystal system). This energy was found to be an optimum for the following reasons: at lower energies strong diffuse scattering was detected, with undesirable blurring effects and, in addition, the efficiency of the detector scintillator is the highest at energies above 50 KeV. However, going to energies higher than 75–80 KeV lead to a lower readability of characters, probably owing to the exceedingly oscillating behaviour of the incoming X-ray wavefront phase at such high energies. Due to the aspect ratio of the beam (5 mm high × 15 cm wide), the sample (16 cm in length) was moved after each scan by a distance equal to the height of the beam, so that the entire sample could be imaged. During each scan, 2,000 radiograms were recorded over 360 degrees, accounting for a total time of 4 min at each step. The total integration time for the entire sample was ~4 h. The CT reconstruction algorithm used was the gold-standard Fourier-filtered back projection, using an open-source, Graphics Processing Unit (GPU)-based implementation of the PyHST2 code [32] . 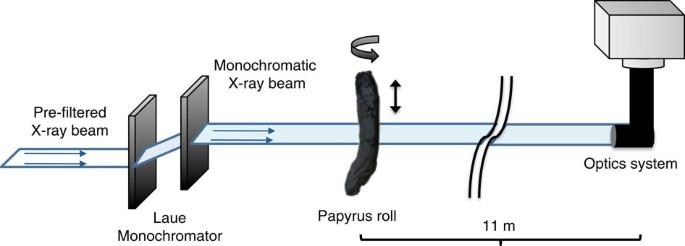Figure 5: The experimental set-up. A pre-filtered synchrotron X-ray wavefront is monochromatized by a double Laue-Laue monochromator. The papyrus sample is fixed to a sample stage and rotates over 360 degrees. Due to the aspect ratio of the beam (5 mm high × 15 cm wide), the sample (16 cm in length) is moved after each scan by a distance equal to the height of the beam. After passing through the sample the X-ray beam is recorded by a FReLoN detector. Figure 5: The experimental set-up. A pre-filtered synchrotron X-ray wavefront is monochromatized by a double Laue-Laue monochromator. The papyrus sample is fixed to a sample stage and rotates over 360 degrees. Due to the aspect ratio of the beam (5 mm high × 15 cm wide), the sample (16 cm in length) is moved after each scan by a distance equal to the height of the beam. After passing through the sample the X-ray beam is recorded by a FReLoN detector. Full size image How to cite this article : Mocella, V. et al. Revealing letters in rolled Herculaneum papyri by X-ray phase-contrast imaging. Nat. Commun. 6:5895 doi: 10.1038/ncomms6895 (2015).